Calix[n]imidazolium as a new class of positively charged homo-calix compounds Macrocycles based on neutral calixarenes and calixpyrroles have been extensively explored for ion binding, molecular assembly and related applications. Given that only these two types of calix compounds and their analogs are available, the introduction of new forms of widely usable calix macrocycles is an outstanding challenge. Here we report the quadruply/quintuply charged imidazole-based homo-calix compounds, calix[4/5]imidazolium. The noncovalent (C-H) + /π + -anion interactions of the imidazolium rings with anions inside and outside the cone are the stabilizing factors for crystal packing, resulting in self-assembled arrays of cone-shaped calix-imidazolium molecules. Calix[4]imidazolium senses fluoride selectively even in aqueous solutions. Calix[5]imidazolium recognizes neutral fullerenes through π + –π interactions and makes them soluble in water, which could be useful in fullerene chemistry. Not only derivatization and ring expansion of calix[ n ]imidazolium, but also their utilization in ionic liquids, carbene chemistry and nanographite/graphene exfoliation could be exploited. Two types of calix compounds, calixarenes and calixpyrroles, have been known for more than a century. Calixarenes have been widely used as ionophores and receptors [1] , [2] , [3] . Their derivatives, including substituted benzene and benzene-like molecules such as calixpyridines, have been extensively explored for intriguing self-assembly of nanoelectronic and nanooptical materials, and various crystal structures exhibiting extraordinary architecture have been reported [4] , [5] , [6] , [7] , [8] , [9] , [10] , [11] , [12] . Calixpyrroles have also been utilized as anion sensors [13] . A number of calixpyrrole-based supramolecules and their analogs including calixfurans, calixthiophenes, calixindoles and calixphyrins have been synthesized and used in diverse applications [14] , [15] , [16] , [17] , [18] . Derivatization, ring expansion and substitution with various functional moieties have been important factors in the advancement of the anion-sensing abilities of calix compounds. Calix molecules, by virtue of their inherent nature, have been extensively explored toward not only the advancement in molecular recognition and supramolecular assembly vis-à-vis crystal engineering, but also toward their application in biological [19] , [20] , [21] and environmental areas [22] including ionophores, extractions and transports [23] , [24] , [25] , [26] . The molecular recognition by the two types of neutral calix compounds is generally based on neutral or charged hydrogen bonds. Neutral hydrogen bonds for anions occur through N-H···anion interaction by amide, pyrrole, urea, ammonium and guanidinium groups. The negatively charged moiety of N or O can provide hydrogen bonds with cations. On the other hand, recently, the (C-H) + ···anion ionic H-bond by the imidazolium group has been explored to synthesize positively charged receptors [27] , [28] , [29] , [30] , [31] , [32] , [33] . Mostly, the reported imidazolium-based receptors have one to four imidazolium moieties in the form of tweezers, dipodal, tripodal and other open forms. Until now, imidazolium-based macrocycles have received less attention than the open-form counterparts, while some examples of imidazolium-based pseudo-calix (or hetero-calix) compounds and cyclophanes have been reported [31] , [34] , [35] , [36] , [37] , [38] , [39] . Utilization of the ionic H-bonding by imidazolium moieties, which is much stronger than the H-bonding of the pyrrole and urea moieties [31] , would improve the binding affinity for the anion. In particular, the design of receptors with an array of positively charged imidazolium moieties in calix form would enhance the binding affinity toward the anions, and the selectivity for anions could be varied depending on the cavity size [40] . However, despite the progress made in the development of imidazolium-based anion receptors in the last decade, a truly imidazolium-based homo-calix compound, analogous to calix[ n ]arene defined as having a [1 n ]metacyclophane skeleton [41] and calix[ n ]pyrrole, is not yet reported. Here, we report the simple one-pot synthesis of quadruply and quintuply positively charged calix[4]imidazolium and calix[5]imidazoium, which have an array of four and five imidazolium moieties connected by methylene bridge, respectively. We investigated the binding affinity for fluoride [40] in aqueous solution. We show that calix[5]imidazolium enables neutral C 60 fullerenes to be soluble in water, and is used to recognize the neutral fullerenes and nanographite/graphene flakes through novel π + –π interaction [42] . In the future, these calix[ n ]imidazolium compounds and their derivatives could be applied in carbene chemistry [43] , [44] , [45] , [46] , [47] as well as in applications requiring novel ionic liquids [48] , [49] . Synthesis and single-crystal X-ray analysis A simple one-pot synthesis provided a new type of positively charged imidazolium-based homo-calix compounds that were observed as a single-crystal structure of calix[4]imidazolium ( I ) in the form of a chloride salt, I ·4Cl·X·H 5 O 2 (X=Cl/Br=0.5Cl·0.5Br) and calix[5]imidazolium ( II ) in the form of a bromide salt, II ·5Br·[F·H 5 O 2 ]. This is the first example of a positively charged imidazolium-based homo-calix compound. We adopted a template-directed synthesis with the chloride and bromide anions in the ring closure reaction to synthesize the calix[4/5]imidazolium receptors [35] , [36] . The anion receptor, [calix[4]imidazolium]-[tetrabromide] ( I ·4Br), was synthesized through the reaction of 1-(1 H -imidazol-1-ylmethyl)-1 H -imidazole and tetrabutylammonium-chloride (TBA-Cl) in dibromomethane (CH 2 Br 2 ), followed by anion exchange with ammonium hexa-fluoro phosphate (NH 4 PF 6 ). Finally, we succeeded in synthesizing the receptor I ·4Cl·X·H 5 O 2 through anion exchange with excess HCl aqueous solution ( Fig. 1 ). The procedure to synthesize I ·4Cl·X·H 5 O 2 was also applied to synthesize II ·5Br with the addition of tetrabutylammonium-bromide (TBA-Br) in the place of TBA-Cl ( Fig. 1 ). Crystals of the anion receptors ( I and II ) were obtained by slow air drying of a water solution. The crystal structures of the anion receptors ( I and II ) were characterized by single-crystal X-ray diffraction analysis ( Supplementary Data 1–3 ) and 1 H-NMR. 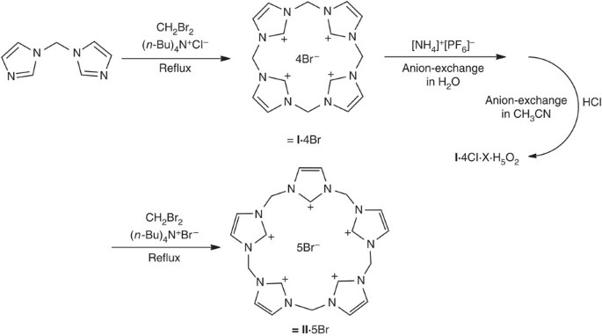Figure 1: Synthesis of I and II. An efficient one-pot synthesis generates a new type of positively charged imidazolium-based calix[n]imidazolium compounds. Figure 1: Synthesis of I and II. An efficient one-pot synthesis generates a new type of positively charged imidazolium-based calix[ n ]imidazolium compounds. Full size image We have isolated a single-crystal structure of I ·4Cl as I ·4Cl·X·H 5 O 2 [= I 4+ ·4Cl − ·X − ·(H 5 O 2 ) + ] ( Fig. 2 ). A quadruply positively charged organic macrocyclic molecule ( I ) in a tetragonal unit cell is surrounded by one X(1), four Cl(2) and one (H 5 O 2 ) + ( Fig. 2a ). The cross sections of planes (220) and (040) in Fig. 2a denote the packing structures of the cone-shaped I ·4Cl·X in Fig. 2b and c , respectively. When the structure is viewed through the b -axis, the cone conformations are arrayed in the same direction ( Fig. 2c ), while piled layers of cone conformations are arranged alternatively in opposite directions ( Fig. 2b ). In the packing pattern, each of the top X(1) of I ·4Cl·X has π + -anion interactions [50] with the quadruply positively charged π-system of the imidazolium moieties in I ·4Cl·X ( Fig. 2b ). While each of the four Cl(2) at the base of the cone conformation of I ·4Cl·X has an extended coordination by forming a CH···Cl − H-bond with a bridging CH 2 group of the second I ·4Cl·X lying below. Four nearby units of I ·4Cl·X surround a positively charged (H 5 O 2 ) + , which is charge-balanced by the neighboring Cl − anions and stabilized by the O-H···Cl − H-bonds. The (H 5 O 2 ) + cation resides on a two-fold rotation axis of the Zündel-type structure (bond distances: O1–H1s (1.172 Å) and O1···O1 a (2.34(1) Å); Fig. 2d ). Altogether, the noncovalent interactions involving the (C-H) + ···Cl − ionic H-bond, the C-H···Cl − H-bonds and the π + -anion interaction of X − with four imidazolium rings are responsible for regular crystal packing toward the formation of an array of the cone-shaped I ·4Cl·X units as a building block, where one chloride/bromide [X(1)] is bound at the top center of the cone and the chloride/bromide [X(1)] ion at the bottom center of the cone. The formation of the relatively small cavity size of the cone could be utilized for the recognition of small anions such as fluoride. 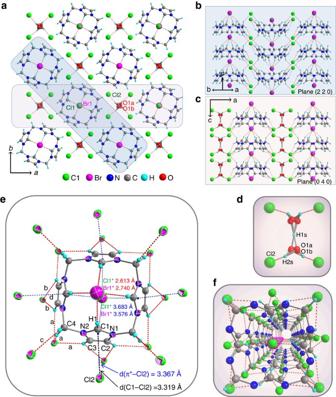Figure 2: X-ray crystal structures of I·4Cl·X·H5O2(X=Cl/Br). (a) The unit cell structure of (I4+·4Cl−·X)−·(H5O2)+viewed along thec-axis. Planes (220) and (040) are represented in shaded boxes. (b) Packing structure of I·4Cl·X·H5O2on the plane (220). (c) Packing structure of I·4Cl·X·H5O2on the plane (040). (d) Structure of (H5O2)+·4Cl−. Dashed lines indicate H-bonds like ionic Cl−···H2O. (e) Structure of [I·4Cl·X]−showing different types of interactions.a=2.680, 2.731, 2.858 Å,b=2.805, 3.136 Å,c=2.686 Å,d=3.367 Å. (f) The perspective structure of arrays of [I·4Cl·X]−. In (b–f), the (C-H)+···X−ionic H-bonds are in thick dashed red lines; π+···Cl−interactions in thick dashed blue lines; CH···Cl−H-bonds in thin dotted red lines. In (a), only the (C-H)+···X−and O-H···Cl−, H-bonds are drawn in red color for visual clarity. As the Cl/Br is alternatively occupied, the corresponding O in H5O2is positioned slightly differently, and so the O position is not given at a single point, but at four different points (O1a, O1b, O1a’, O1b’ ind) close to each other; otherwise, a supercell needs to be used. Figure 2: X-ray crystal structures of I·4Cl·X·H 5 O 2 (X=Cl/Br). ( a ) The unit cell structure of (I 4+ ·4Cl − ·X) − ·(H 5 O 2 ) + viewed along the c -axis. Planes (220) and (040) are represented in shaded boxes. ( b ) Packing structure of I·4Cl·X·H 5 O 2 on the plane (220). ( c ) Packing structure of I·4Cl·X·H 5 O 2 on the plane (040). ( d ) Structure of (H 5 O 2 ) + ·4Cl − . Dashed lines indicate H-bonds like ionic Cl − ···H 2 O. ( e ) Structure of [I·4Cl·X] − showing different types of interactions. a =2.680, 2.731, 2.858 Å, b =2.805, 3.136 Å, c =2.686 Å, d =3.367 Å. ( f ) The perspective structure of arrays of [I·4Cl·X] − . In ( b – f ), the (C-H) + ···X − ionic H-bonds are in thick dashed red lines; π + ···Cl − interactions in thick dashed blue lines; CH···Cl − H-bonds in thin dotted red lines. In ( a ), only the (C-H) + ···X − and O-H···Cl − , H-bonds are drawn in red color for visual clarity. As the Cl/Br is alternatively occupied, the corresponding O in H 5 O 2 is positioned slightly differently, and so the O position is not given at a single point, but at four different points (O1a, O1b, O1a’, O1b’ in d ) close to each other; otherwise, a supercell needs to be used. Full size image As seen in Fig. 2b , c and e , the receptor I forms a cone conformation of all four imidazolium (C-H) + moieties whose (C-H) + groups point toward the top X(1) and whose rings face toward the bottom X(1). Thus, X(1) is octa-coordinated by four (C-H) + ···X − ionic H-bonds and four π + ···X − π + -anion interactions. The distance from a H-atom of the imidazolium (C-H) + group to the top X(1) Cl − /Br − is 2.613/2.740 Å, while the distances from the bottom X − to the centroid of the positively charged imidazolium ring and the positively charged C atom in the (C-H) + group are 3.683/3.576 Å and 4.006/3.859 Å, respectively ( Fig. 2e ). Sixteen chloride atoms (Cl(2)) are located outside the cage of I with the aid of CH···Cl − H-bonds and the π + ···Cl − interaction, and these interaction distances are denoted as a – d in Fig. 2e : each of four Cl(2) anions is coordinated with the 3-H of an imidazolium moiety, the 4-H of the bridging CH 2 group and the 3-H of an adjacent imidazolium moiety at a distance of 2.680–2.858 Å, b : each of four Cl(2) anions is coordinated with the 2-H and 3-H of an imidazolium moiety at a slightly longer distance (2.805–3.136 Å), c : another four Cl − anions are each coordinated with the second 4-H of the bridging CH 2 group in I at a distance of 2.686 Å, and d : each of four Cl − anions forms a π + -anion interaction individually with the positively charged π-system of imidazolium moieties of I at the distance of 3.367 Å from the carbon atom of the (C-H) + group. Each imidazolium moiety is hepta-coordinated with the top X(1) ((C-H) + ···X − ionic H-bond at the distance of 2.613/2.740 Å), the bottom X(1) (π + ···X − interaction at the distance of 3.683/3.576 Å), the Cl(2) (π + ···Cl − interaction at the distance of 3.367 Å) and the four CH···Cl − (2) interactions. Each of the Cl(2) anions has octa-coordination by six H-bonds surrounding the imidazolium moieties of I , one H-bond with (H 5 O 2 ) + , and one π + ···anion interaction. The cone conformations of I ·4Cl·X·H 5 O 2 are stacked one above another continuously. This stacked structure results in a one-dimensional Cl − array inside each pore comprising cavities ( Fig. 2f ) of stacked calix compounds. The isolated crystal structure of the quintuply positively charged organic macrocyclic molecule ( II ) also adapted a cone conformation. It is composed of five different imidazoles connected through a methyl carbon. As in Fig. 3 , the calix[5]imidazolium ( II ) has two types of interaction with the bromide anion that is located almost at the center of the cavity in this host molecule. The ionic H-bond interaction has three different distances from bromide to the hydrogen of imidazole (C-H) + , 3.242 Å toward H2, 3.684 Å toward H6 and 3.307 Å toward H10. The other interaction is π + ···Br − interaction between the imidazolium moiety and the bromide anion, which is an edge-to-face mode. Each of these three π + ···Br − interactions have distances of 3.711 Å, 3.541 Å and 3.708 Å, respectively. These interactions stabilize the calix structure with a bromide anion centered in the cavity. 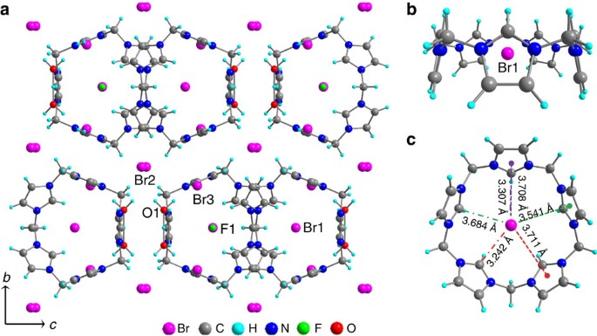Figure 3: X-ray crystal structures of II·5Br·[F·H5O2]. (a) The unit cell structure viewed along thea-axis. A unit cell is denoted by a red box. (b). Side and top views of the structure of II·5Br·[F·H5O2] showing the (C-H)+···Br−ionic H-bonds in thick dashed and dotted red line for Br1-H2, in green line for Br1-H6, and in violet line for Br1-H10, where the interactions are shown in thick dashed lines from the bromide anion to the centroid of an imidazole moiety. Figure 3: X-ray crystal structures of II·5Br·[F·H 5 O 2 ]. ( a ) The unit cell structure viewed along the a -axis. A unit cell is denoted by a red box. ( b ). Side and top views of the structure of II·5Br·[F·H 5 O 2 ] showing the (C-H) + ···Br − ionic H-bonds in thick dashed and dotted red line for Br1-H2, in green line for Br1-H6, and in violet line for Br1-H10, where the interactions are shown in thick dashed lines from the bromide anion to the centroid of an imidazole moiety. Full size image Water-soluble fullerene using calix[5]imidazolium (II) Given the strong π + –π interaction that has been explored in molecular recognition [42] , a bowl-shaped structure of calix[5]imidazolium led us to expect detection of fullerenes in aqueous solution. The spectroscopic results of fluorescence and NMR indicate that a boiling aqueous solution of II ·5Br provides water-soluble fullerene ( Supplementary Fig. S17 – S19 ), which would be very useful for fullerene science. The fluorescence emission spectrum of C 60 in an aqueous solution of II ·5Br showed an intensity enhancement, indicating the strong interaction between the calix[5]imidazolium (π + ) and fullerene (π) systems. The chemical shift of the carbon in calix[5]imidazolium shows that the interaction takes place at the double bond of the imidazolium ring, not the (C-H) + moiety of imidazolium. Every carbon in calix[5]imidazolium shifted downfield except for the carbon of imidazolium (C-H) + , while the characteristic single signal of fullerene in water was also observed. These results, which show an agreement with the calculated geometries ( Supplementary Fig. S20 ), provide evidence for the interaction of the fullerene carbon cage and calix[5]imidazolium, as an important example of π + –π interaction contribution to the sensing process. Recognition of aqueous fluoride by calix[4]imidazolium (I) To understand the binding features, we carried out isothermal titration calorimetry I ·4Cl·X·H 5 O 2 toward the fluoride anion in aqueous solution at room temperature. The binding isotherm curve fitted the one-site model indicating a 1:1 complexation with a large binding constant of 8.3 × 10 4 M −1 (average value), as shown in Fig. 4 and Supplementary Fig. S1 . 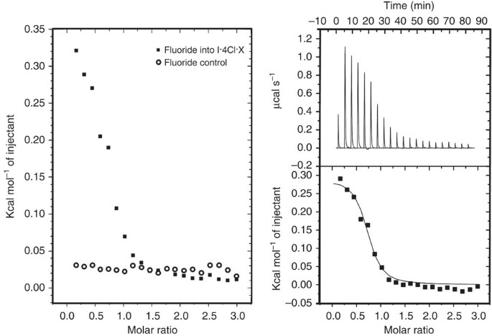Figure 4: Isothermal titration calorimetry (ITC) data of 0.5 mM I·4Cl·X·H5O2(=I·4Cl·X ) in H2O with 10 mM tetrabutylammonium fluoride (TBA-F). Left: ITC ΔH of 10 μl injection of 10 mM TBA-F into 0.5 mM I·4Cl·X·H5O2in water, experimental data (▪) and control data (○). Right: ITC thermogram of TBA-F into I·4Cl·X·H5O2. Figure 4: Isothermal titration calorimetry (ITC) data of 0.5 mM I·4Cl·X·H 5 O 2 (=I·4Cl·X ) in H 2 O with 10 mM tetrabutylammonium fluoride (TBA-F). Left: ITC ΔH of 10 μl injection of 10 mM TBA-F into 0.5 mM I·4Cl·X·H 5 O 2 in water, experimental data (▪) and control data ( ○ ). Right: ITC thermogram of TBA-F into I·4Cl·X·H 5 O 2 . Full size image In a single-crystal structure, a unit cell includes an excess chloride and one (H 5 O 2 ) + ion. Thus, to investigate the influence of chloride, we prepared neutral I ·4Cl by anion exchange with ammonium chloride (NH 4 Cl). The calorimetric titration of this neutral I ·4Cl still provided a large binding affinity of 2.5 × 10 4 M −1 , though slightly smaller than the case of I ·4Cl·X·H 5 O 2 , which implies that the excess chloride does not have a significant effect on the binding affinity toward F − . Additionally, the calorimetric titration of neutral I ·4Cl with F − in a slightly acidic buffered solution (where the neutral I ·4Cl was tuned to the 6.04 pH value with a 50 mM 2-(N-morpholino) ethanesulfonic acid (MES)/NaOH buffer solution, which has a similar pH to that of I ·4Cl·X·H 5 O 2 ) showed a titration curve very similar to the case of I ·4Cl·X·H 5 O 2 . Finally, the calorimetric titrations of I ·4Br − toward F − provided a binding constant of 1.78 × 10 4 M −1 , which is still close to that of I ·4Cl·X·H 5 O 2 with F − (1.81 × 10 4 M −1 ) in the presence of Br − (in the form of TBA-Br). Therefore, the presence of excess chloride/bromide or other counter anions or protons does not have a significant effect on the binding of I with F − ( Supplementary Fig. S2–5 and Supplementary Table S1 ). Furthermore, we checked the 19 F-NMR chemical shift changes of fluoride (TBA-F in D 2 O) upon interacting with I ·4Cl·X·H 5 O 2 , 1:1 molar ratio ( Supplementary Fig. S6 ). The peak at −122.5 p.p.m. of the 10 mM TBA-F in D 2 O slightly changed to −127 p.p.m. upon the addition of 1 molar equivalent of I ·4Cl·X·H 5 O 2 . In addition, a new signal appeared at −147 p.p.m. due to the complexation of F − with the receptor. Finally, the analysis of positive/negative electrospray ionization mass spectrometry suggested the presence of 1:1 binding mode between I ·4Cl·X·H 5 O 2 and fluorides ( Supplementary Fig. S8 ). Variable-temperature NMR studies were performed to investigate possible conformers in solution for both I and II as Br − and PF 6 − salts. Our variable-temperature NMR studies were done in the temperature ranges of 25 to 90 °C for Br − salts in water (as Br − salt is soluble only in water) and −40 to 75 °C for PF 6 − salts in acetonitrile:water (5:1) solvent mixture ( Supplementary Fig. S25–28 ). In both cases, it seems that only one conformer is present in the solution over a wide range of temperatures; however, which form of the conformer would be present could not be rationalized from the NMR data. We further attempted to correlate this data with the crystal data. We were able to isolate the crystal structure of an 1,2-alternate conformer of I in the presence of counterion (Br − ), unlike the observation of cone conformer obtained with excess counterion (Cl − ) (due to HCl that was required for crystallization of the host). On the other hand, the 1,2-alternate conformer of I ·4Br is different from the cone conformer of II ·5Br salt observed in the crystal structure. For I or II , the existence of alternate and cone-conformers in solution or crystal depending on the counteranion seem to be controlled by the effectiveness in the ion-pair interaction between the host and Cl − /Br − /PF 6 − anions ( Supplementary Fig. S24 : description). Calix[4]imidazolium is able to make N-heterocyclic carbene (NHC) complexes. Silver complexes of NHC show antimicrobial activity [47] and are used as NHC transfer agents in transition metal chemistry [46] . As a preliminary study, we identified the silver carbene complex of calix[4]imidazolium using 1 H-NMR and 13 C-NMR ( Supplementary Fig. S9 ). Theoretical calculations To understand the conformational structures of I ·4Cl, I ·4Br, [ I ·5Cl] − and [ I ·4Cl·F] − , we performed density functional theory (DFT) calculations (BLYP/6-31+G* level) for important conformational structures including two types of cone-conformers (c and t; c: one X − is respectively coordinated from top and bottom of the cone, t: only one X − is coordinated from the top of the cone), 1,2 and 1,3-alternate conformers (a12 and a13, respectively), and partial cone conformer (p) ( Fig. 5 , Supplementary Fig. S14 and Supplementary Table S7 ). The self-consistent reaction field- polarizable continuum model was used for the calculations in water. For I ·4Cl, the most stable structure is I ·4Cl-c in the gas phase, but I ·4Cl-t in water ( Fig. 5 ). In the cone conformer I ·4Cl-c, one Cl − is bound at the top of the cone with (C-H) + ···Cl − ionic H-bonds and another Cl − is bound at the bottom of the cone with the π + -anion interaction. In the I ·4Cl − -t conformer, one Cl − is bound at the top of the cone with (C-H) + ···Cl − ionic H-bonds and other three Cl − anions are bound below with multiple CH···Cl − H-bonds. 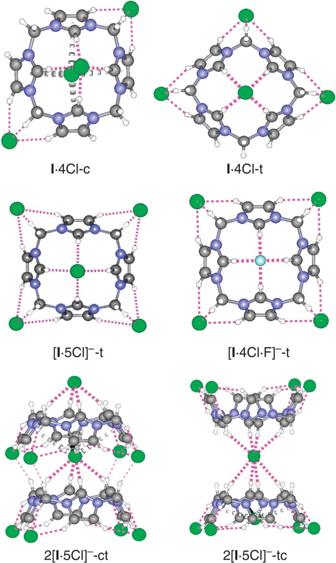Figure 5: B3LYP self consistent reaction field (SCRF) polarizable continuum model (PCM) optimized geometries of the cone-conformers of I·4Cl-c/t, [I·5Cl]−-t, [I·4Cl·F]−-t, 2[I·5Cl]−-ct and 2[I·5Cl]−-tc. The (C-H)+···Cl−ionic H-bonds and CH···F−/Cl−H-bonds are denoted by red dotted lines (distance ~2.7 Å or less); π+-anion interactions between Cl−and positively charged imidazolium rings are in gray dotted lines. In aqueous solvent, (H5O2)+would not be present, so the water surrounding [I·5Cl]−was taken into account with SCRF PCM calculations. Figure 5: B3LYP self consistent reaction field (SCRF) polarizable continuum model (PCM) optimized geometries of the cone-conformers of I·4Cl-c/t, [I·5Cl] − -t, [I·4Cl·F] − -t, 2[I·5Cl] − -ct and 2[I·5Cl] − -tc. The (C-H) + ···Cl − ionic H-bonds and CH···F − /Cl − H-bonds are denoted by red dotted lines (distance ~2.7 Å or less); π + -anion interactions between Cl − and positively charged imidazolium rings are in gray dotted lines. In aqueous solvent, (H 5 O 2 ) + would not be present, so the water surrounding [I·5Cl] − was taken into account with SCRF PCM calculations. Full size image For [ I ·5Cl] − , the cone conformer [ I ·5Cl] − -t, which is constructed by adding additional Cl − in the I ·4Cl-t conformer, is the most stable conformer both in the gas phase and in water. For the binding mode of F − with I ·4Cl, the cone conformer [ I ·4Cl·F] − -t is much more stable than other conformers both in the gas phase and in water. Therefore, the 1:1 binding pattern of [ I ·4Cl·F] − upon formation of complexes with I ·4Cl or [ I ·5Cl] − would be the cone form; for the latter case, one of the Cl − would be replaced by the incoming F − anion. We also investigated the intriguing crystal packing in I ·4Cl·Cl·(H 5 O 2 ) with DFT calculations (RI-B3LYP/TZVP level) for various structures of [ I ·5Cl] − , 2[ I ·5Cl] − , 3[ I ·5Cl] − and 4[ I ·5Cl] − ( Supplementary Fig. S15 and Supplementary Table S8 ). The COnductor-like Screening MOdel (COSMO) was used to treat the aqueous phase. As [ I ·5Cl] − -t is the most stable conformer, it is conceivable that during crystal packing this conformer would have the most significant role apart from other important interaction involving the H 5 O 2 + moiety. As one [ I ·5Cl] − -t approaches from below or top to another conformer, it would form the dimer 2[ I ·5Cl] − -ct ( Supplementary Fig. S15 ) in which one of the Cl − in between the two imidazolium rings is bound by four (C-H) + ···Cl − ionic H-bonds from below and by the π + -anion interaction with four positively charged imidazolium rings from above. Another form of the dimer, 2[ I ·5Cl] − -tc, where one Cl − has eight (C-H) + ···Cl − ionic H-bonds from two oppositely faced calix[4]imidazolium, is unlikely to form as it is much less stable than the 2[ I ·5Cl] − -ct dimer ( Fig. 5 , Supplementary Fig. S15 ). Subsequent packing of [ I ·5Cl] − -t either from above or below the 2[ I ·5Cl] − -ct dimer would lead to the formation of the trimer (3[ I ·5Cl] − -2ct) ( Supplementary Fig. S15 ). Further associations of a trimer or of two dimers would form the tetramer of 4[ I ·5Cl] − -3ct. Hence, step by step associations of monomers/n-mers of [ I ·5Cl] − -t would elongate the packing to the infinite length, whereby each of the [ I ·5Cl] − -t represents the building block of the crystal packing toward an infinite length of an array of cones. We have also carried out the possible structures of II·5Br interacting with the neutral C 60 fullerene using resolution identity-DFT ( Supplementary Fig. S20 ). The most stable structure is depicted in Fig. 6 . The C 60 fullerene matches well with the cavity size formed by five imidazole rings of II . The structure clearly shows the strong stacked π + –π interactions between the positively charged five imidazolium rings (π + ) and the aromatic fullerene carbon cage (π). When the (C-H) + groups of imidazole rings interact with the fullerene cage, the structure is much less stable ( Supplementary Fig. S20 ). This also explains why the fullerene is soluble in water by interaction with highly positively charged calix[5]imidazolium. 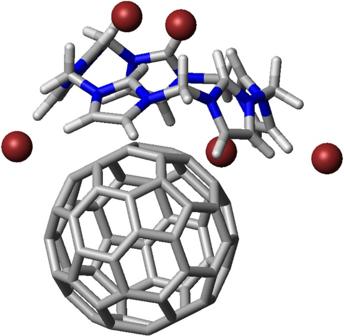Figure 6: The most stable geometry of the complex composed of the neutral C60fullerene and II·5Br. Calculations were carried out with resolution identity-DFT. Figure 6: The most stable geometry of the complex composed of the neutral C 60 fullerene and II·5Br. Calculations were carried out with resolution identity-DFT. Full size image We have synthesized the first quadruply positively charged homo-calix compound, calix[4]imidazolium in the form of a chloride salt ( I ·4Cl·X·H 5 O 2 ). It has four positively charged imidazolium moieties to form a macrocycle connected through methyl bridges. The single X-ray crystal structure of [ I ·4Cl·X·H 5 O 2 ] elucidated that it had a cone-like conformation with all four imidazolium (C-H) + groups pointing towards one chloride ion at the top of the center in the cavity, while their faces interacted with another chloride ion at the bottom in the cavity. The noncovalent interactions, that is, (C-H) + ···Cl − ionic H-bond, CH···Cl − H-bonds, OH···Cl − H-bonds and π + -anion interactions of Cl − with four imidazolium rings of I from inside and outside of the cone, caused the crystal growth of negatively charged ( I ·4Cl·X) − and positively charged (H 5 O 2 ) + of infinite length. This receptor displays excellent binding affinity for F − in aqueous media revealing 1:1 binding stoichiometry between F − and I ·4Cl·X·H 5 O 2 , which was demonstrated by isothermal titration calorimetry and DFT calculations. Molecular assembly phenomena utilizing calix[ n ]imidazolium as the building blocks by utilizing various forms of neutralizing counter anions should open a challenging task in crystal engineering. We also synthesized an expanded ring compound, calix[5]imidazolium, which has a larger cavity size than calix[4]imidazolium, and characterized its X-ray structure. This expanded ring allows recognition of larger-size anions through electrostatic interactions. Importantly this calix[5]imidazolium enables neutral C 60 fullerenes soluble in water, and is used to recognize neutral fullerenes through novel π + –π interactions, which have hardly been utilized in supramolecular chemistry. This interaction has been demonstrated by fluorescence and NMR spectroscopy as well as by theoretical calculations of the calix[5]imidazolium and fullerene complex. Eventually, this recognition could be utilized to diverse aromatic systems such as DNA bases, proteins and nanographite/graphene flakes ( Supplementary Fig. S21 ). Therefore, these are indeed significant findings with possible wide applications in many branches of science. Additionally, the synthesis of other forms of calix[ n ]imidazolium receptors by means of derivatization, incorporation with chromo/fluorogenic moieties, hydrophobic tails and expanded rings, ( Supplementary Fig. S22 ) as well as its utilization in ionic liquids ( Supplementary Fig. S23 ) and carbene chemistry should open a new field in supramolecular chemistry. General procedures and synthesis Imidazole, dibromomethane and tetrabutylammonium fluoride/chloride were purchased from Aldrich. 1 H-NMR and 13 C-NMR spectra was performed on a Bruker Avance DPX500 (Bruker) (500 MHz) spectrometer at 298 K. 19 F-NMR spectra were recorded on a Bruker Avance DPX300 (300 MHz) spectrometer at 298 K. VT 19 F-NMR spectra were carried out on a Bruker Avance DPX500 (500 MHz) at 278, 298, 323, and 343 K. Electrospray ionization mass spectrometry spectra were recorded on a Agilent 6224 TOF LC/MS (Agilent). [Calix[4]imidazolium][pentachloride], I·4Cl·X·H 5 O 2 was synthesized as follows. Dibromomethane (10 ml, 9.79 mmol), 1-(1 H -imidazol-1-ylmethyl)-1 H -imidazole (3.5 mmol, 0.5 g) and tetrabutylammonium-chloride (7.2 mmol, 2 g) were mixed and the reaction mixture was stirred for 30 min. After stirring, the mixture was heated under reflux for 6 h. After cooling to room temperature, the precipitate was isolated and washed with fresh acetonitrile. The precipitate was dissolved in water (1 ml) and a saturated solution of ammonium hexa-fluoro phosphate (NH 4 PF 6 ) (2 ml) was added to the solution. The resulting white precipitate was filtered off and washed with water. The product [calix[4]imidazolium][PF 6 ] 4 dissolved in acetonitrile was ion-exchanged with 12 N HCl solution. The obtained white-colored final product ( I ·4Cl·X·H 5 O 2 ) was recrystallized from water with a yield of 78.7%; 1 H-NMR (500 MHz, D 2 O, 25 °C) δ 9.95 (s, 4H, imidazolium ring -N-C H -N-), δ 8.04 (s, 8H, imidazolium ring -N-C H -C H -N-), δ 6.92 (s, 8H, -N-C H 2 -N-); 13 C-NMR (500 MHz, D 2 O) δ 59.81, 123.95, 139.56. For the synthesis of [Calix[5]imidazolium][pentabromide] ( II ·5Br − ), 1-(1 H -imidazol-1-ylmethyl)-1 H -imidazole (3.5 mmol, 0.5 g) and tetrabutylammonium-bromide (7.7 mmol, 2.5 g) were added to dibromomethane (10 ml, 9.79 mmol), and the mixture was stirred for 30 min. After stirring, the mixture was heated under reflux for 6 h. After cooling to room temperature, the precipitate was isolated and washed with fresh acetonitrile. The final white-colored product was recrystallized from water with a yield of 75.3%; 1 H-NMR (500 MHz, D 2 O, 25 °C) δ 9.99 (s, 5H, imidazolium ring-N-C H -N-), δ 8.07 (s, 10H, imidazolium ring-N-C H -C H -N-), δ 6.94 (s, 10H, -N-C H 2 -N-); 13 C-NMR (500 MHz, D 2 O) δ 59.51, 123.64 and 139.47. Fluorescence measurement Fluorescence measurements were carried out at room temperature. The fluorescence emission spectra were performed with an aqueous solution of II ·5Br (24.8 mM, 10 ml) in the presence of fullerene (0.001 g, 1.38 μmol), by monitoring the change in the intensity of fluorescence emission spectra. The fluorescence emission spectra were obtained using 389 nm excitation. 19 F-NMR measurement Fluorine NMR measurements were carried out at 298 K. The change in chemical shift of the solutions of 10 mM and 2 mM TBA-F in D 2 O upon adding 1:1 molar equivalent of I ·4Cl·X·H 5 O 2 in D 2 O were recorded. The measurements were repeated at least twice to obtain consistent values. For the VT 19 F-NMR, we prepared a 1:1 molar ratio of 250 mM I ·4Cl·X·H 5 O 2 and 10 mM TBA-F, which were monitored at 278 K, 298 K, 323 K and 343 K, respectively. Isothermal titration calorimety Every calorimetric titration was carried out using a fluoride control before titration of the calix[4]imidazolium receptor with respect to fluoride. The calorimetric titrations were repeated at least twice to obtain consistent values. For the calorimetric titrations of I ·4Cl·X·H 5 O 2 and I ·4Br, we prepared 0.5 mM of each calix in water, and 10 mM TBA-F in water was added. For the titration of I ·4Cl, we prepared 1.0 mM I ·4Cl and 10 mM TBA-F in water as a starting concentration. For the case of I ·4Cl in the presence of buffer solution, we prepared 50 mM 2-(N-morpholino)ethanesulfonic acid (MES) buffer solution whose pH was 6.04 by manipulation with sodium hydroxide (NaOH). This MES buffer solution was used to make 0.5 mM of I ·4Cl and 10 mM TBA-F in a 50 mM MES buffer solution. For a competition study of halide anions, the calorimetric titration was carried out by adding 20 mM TBA-F into 1.0 mM I ·4Cl in the presence of 1.0 mM TBA-Br. Theoretical calculations The details of DFT calculation results are provided in the Supplementary Information . Accession codes: The Cambridge Crystallographic Data Center ( http://www.ccdc.cam.ac.uk/conts/retrieving.html ) hosts the crystallographic data for these compounds. The single-crystal diffraction data for I·4Cl·X·H 5 O 2 , II ·5Br, and I ·4Br were deposited as CCDC-740391, CCDC-836759, and CCDC-916190 respectively. How to cite this article: Chun, Y. et al . Calix[ n ]imidazolium as a new class of positively charged homo-calix compounds. Nat. Commun. 4:1797 doi: 10.1038/ncomms2758 (2013).